Conclusive quantum steering with superconducting transition-edge sensors Quantum steering allows two parties to verify shared entanglement even if one measurement device is untrusted. A conclusive demonstration of steering through the violation of a steering inequality is of considerable fundamental interest and opens up applications in quantum communication. To date, all experimental tests with single-photon states have relied on post selection, allowing untrusted devices to cheat by hiding unfavourable events in losses. Here we close this 'detection loophole' by combining a highly efficient source of entangled photon pairs with superconducting transition-edge sensors. We achieve an unprecedented ∼ 62% conditional detection efficiency of entangled photons and violate a steering inequality with the minimal number of measurement settings by 48 s.d.s. Our results provide a clear path to practical applications of steering and to a photonic loophole-free Bell test. Quantum entanglement enables unconditionally secure communication and powerful devices such as quantum computers. In their strongest form, the correlations associated with entanglement rule out locally causal world views via tests of Bell inequalities [1] . In a weaker regime, quantum correlations can still be harnessed to steer quantum states, demonstrating that two parties, Alice and Bob, share entanglement even if one party is untrusted [2] . Quantum steering was originally introduced by Erwin Schrödinger [3] , in reaction to the Einstein, Podolsky and Rosen (EPR) 'paradox' [4] ; it describes the ability to remotely prepare different ensembles of quantum states by performing measurements on one particle of an entangled pair, demonstrating the paradox. Depending on the measurement and its random outcome, the remote system is prepared in a different state; however, the unconditioned remote state remains unaffected, thus preventing any possible superluminal signalling. Interestingly, steering and Heisenberg's uncertainty principle have recently been linked to Bell non-locality [5] . The original form of the EPR paradox was demonstrated experimentally with atomic ensembles [6] , continuous-variable states of light [7] , [8] and position-momentum entangled single photons [9] . More recently, quantum steering was redefined in a quantum information context in ref. 2 , promising new applications such as quantum communication using untrusted devices [10] . This new formalization also allows a strict comparison between the concepts of Bell non-locality, steering and entanglement [2] : Bell non-locality requires steering, which in turn requires entanglement. In analogy to entanglement witnesses [11] and Bell inequalities [12] , one can derive experimental criteria [13] to demonstrate steering: steering inequalities impose limits on the observable correlations that can be explained without the need to invoke quantum steering. An experimental violation of a steering inequality was recently reported in ref. 14 . Steering—in a more general sense—has also been shown to be one of two contributors to the degree of Bell non-locality, the other being the uncertainty principle [5] . In this sense, there can be perfect steering in both quantum mechanics and in local hidden-variable theories—their uncertainty relations dictate their different degrees of non-locality. We demonstrate here states with high steerability, in contrast to states in deterministic classical mechanics that have no uncertainty and no steerability. 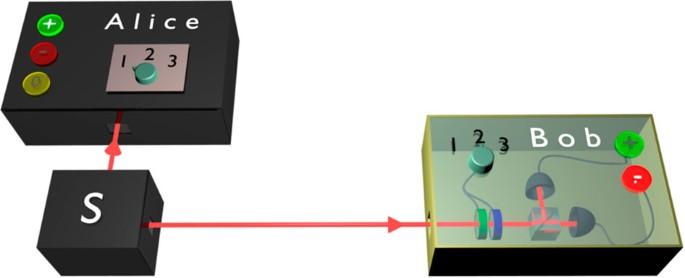Figure 1: Conceptual depiction of quantum steering. Alice and Bob receive particles from a black box (the source,S) and want to establish whether these are entangled. From a prearranged set, they each choose measurements to be performed on their respective particles. Bob's measurement implementation is trusted, but this need not be the case for Alice's; her measurement device is also treated as a black box from which she gets either a 'conclusive',Ai=±1, or a 'non-conclusive' outcome,Ai=0. To demonstrate entanglement, Alice and Bob need to show that she can steer his state by her choice of measurement. They can do so through the violation of a steering inequality: whenever Bob's apparatus detects a particle, Alice needs to provide her measurement result. If the recorded correlations of their measurement results surpass the bound imposed by the steering inequality, Alice and Bob have conclusively proven the entanglement of their particles. We define the steering task in Figure 1 : Alice and Bob receive quantum states from a source and measure them using randomly chosen measurements from a prearranged set; if the observed correlations violate a steering inequality, then Alice and Bob will be convinced that their shared states were entangled. This holds true even if Alice and Bob trust neither the source nor Alice's measurement device. Figure 1: Conceptual depiction of quantum steering. Alice and Bob receive particles from a black box (the source, S ) and want to establish whether these are entangled. From a prearranged set, they each choose measurements to be performed on their respective particles. Bob's measurement implementation is trusted, but this need not be the case for Alice's; her measurement device is also treated as a black box from which she gets either a 'conclusive', A i =±1, or a 'non-conclusive' outcome, A i =0. To demonstrate entanglement, Alice and Bob need to show that she can steer his state by her choice of measurement. They can do so through the violation of a steering inequality: whenever Bob's apparatus detects a particle, Alice needs to provide her measurement result. If the recorded correlations of their measurement results surpass the bound imposed by the steering inequality, Alice and Bob have conclusively proven the entanglement of their particles. Full size image Similarly to the case of Bell inequalities, a conclusive violation of a steering inequality requires that the experiment does not suffer from any relevant loopholes. When one party has untrusted equipment, the so-called detection loophole [15] in particular is critical: if Alice and Bob have to post select their data on Alice's detected events, then low efficiencies enable her measurement devices to cheat by dropping unfavourable results—in the context of quantum key distribution, for instance, this would allow the untrusted supplier of the devices to access the key. The fair sampling assumption invoked in ref. 14 , for instance, is not satisfactory for such untrusted devices. Here we close the detection loophole by using an entangled photon source with high pair collection efficiency [16] , [17] and highly efficient transition-edge sensors (TESs) [18] . We test a steering inequality that naturally accounts for Alice's non-detected events, and violate it by at least 48 standard deviations with the minimum number of two measurement settings and by more than 200 standard deviations for measurements in three different bases. A quadratic steering inequality for qubits To demonstrate steering, Alice and Bob need to be able to freely choose and perform different measurements; we consider the case where each of them can perform N =2 or 3 measurements, labelled i , j= 1,2 or 3, with a priori binary outcomes A i , B j =±1 as shown in Figure 1 . As Bob trusts his measuring device his measurement can be described by a well-characterized quantum observable B̂ j . He considers only the cases where his measurement gives him a conclusive result, that is, when at least one of his detectors clicks—if both click, Bob outputs a random result. In contrast, Alice's devices are not trusted and her measurement apparatus is considered a black box, which is polled whenever Bob receives a result. It returns outcomes A i =±1, indicating conclusive measurement results, or A i =0 when no or both detectors fire. Alice must output a result whenever Bob registers an event, thus any of her inconclusive results cannot be discarded from further analysis. The correlation observed by Alice and Bob can be described by the probability distribution P ( A i = a , B j = b ), with a =±1 or 0, and b =±1. If Bob receives a state that is not entangled to Alice's the set of possible correlations will be restricted, as shown below. First, we define Bob's expectation value for a measurement conditioned on Alice's result, measuring the amount that her results steer his outcomes: Averaging 〈 B 〉 i 〉 A i = a over Alice's results, we define Bob's average expectation As shown in the Methods section, if the correlation P could be explained by the source sending Bob an unentangled two-level system (qubit)—that is, in the terminology of ref. 2 , if the correlation admits a 'local hidden state' model—and if Bob implements qubit measurements in N =2 or 3 mutually unbiased bases, for instance of the Pauli , Ŷ and Ẑ operators, then the following steering inequality holds: where S N is the steering parameter for N bases. Note that the upper bound above depends crucially on Bob's measurement settings, which in experimental implementation will not be perfectly orthogonal, nor perfectly projective; we detail in the Methods section how the bound must be corrected to account for experimental imperfections. Quantum mechanics allows a violation of inequality (3), which thus implies steering. To get a first insight, suppose that Alice and Bob share Werner states of visibility V , where is the Bell singlet state, and that Alice implements the same measurements as Bob. Then, due to the anti-correlation of the singlet state when measured in the same basis, this illustrates that Alice can steer Bob's state to be aligned with her measurement axis, limited by the visibility of the shared state. If Alice has a probability η of getting a conclusive outcome whenever Bob gets one, then This means that the steering inequality (3) will be violated if Satisfying the requirements given by equation (4) in a photonic architecture is challenging. For the minimal set of N =2 measurement settings, an experimental test of the steering inequality (3) requires, even for a pure entangled singlet state with visibility V =1, that Alice detects a signal more than η >50% of the times Bob requests a response. To reach these requirements, the experimental apparatus has to be carefully optimized. 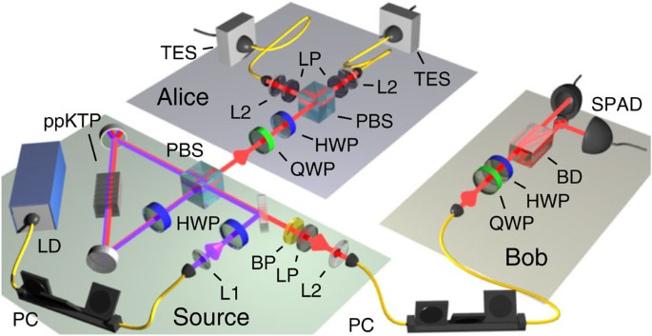Figure 2: Experimental scheme. Polarization-entangled two-photon states are generated in a periodically poled 10 mm KTiOPO4(ppKTP) crystal inside a polarization Sagnac loop16,17. The continuous wave, grating-stabilized 410-nm pump laser (LD) is focussed into this crystal with an aspheric lens (L1,f=4.0 mm) and its polarization is set with a fibre polarization controller (PC) and a half-wave plate (HWP), controlling the entangled output state16. Bob filters his output photon with a long-pass glass filter (LP) and a 3-nm band-pass filter (BP), before collecting it with an aspheric lens (L2,f=18.4 mm) into a single-mode fibre. He performs his measurement in an external fibre bridge, with a combination of a quarter-wave plate (QWP), HWP, a polarizing beam displacer (BD) and multi-mode-fibre-coupled single-photon avalanche diodes (SPADs). To minimize loss, Alice performs her measurement directly at the source using a QWP, HWP and a polarizing beamsplitter (PBS), followed by a LP filter and fibre collection with focussing optics identical to Bob's, finally detecting her photons with highly efficient superconducting transition-edge sensors (TESs)18. Experimental setup We performed our experiment using entangled photons created in a polarization Sagnac source based on spontaneous parametric downconversion [16] , [17] , see Figure 2 . This source design meets two crucial requirements; a high entangled-pair collection efficiency and near-ideal polarization entanglement. Figure 2: Experimental scheme. Polarization-entangled two-photon states are generated in a periodically poled 10 mm KTiOPO 4 (ppKTP) crystal inside a polarization Sagnac loop [16] , [17] . The continuous wave, grating-stabilized 410-nm pump laser (LD) is focussed into this crystal with an aspheric lens (L1, f =4.0 mm) and its polarization is set with a fibre polarization controller (PC) and a half-wave plate (HWP), controlling the entangled output state [16] . Bob filters his output photon with a long-pass glass filter (LP) and a 3-nm band-pass filter (BP), before collecting it with an aspheric lens (L2, f =18.4 mm) into a single-mode fibre. He performs his measurement in an external fibre bridge, with a combination of a quarter-wave plate (QWP), HWP, a polarizing beam displacer (BD) and multi-mode-fibre-coupled single-photon avalanche diodes (SPADs). To minimize loss, Alice performs her measurement directly at the source using a QWP, HWP and a polarizing beamsplitter (PBS), followed by a LP filter and fibre collection with focussing optics identical to Bob's, finally detecting her photons with highly efficient superconducting transition-edge sensors (TESs) [18] . Full size image We followed ref. 17 in the basic design of our source. To maximize the conditional coupling between Alice and Bob's collection apparatus, we optimized the pump and collection spots based on ref. 19 , with the optimum found at using pump spot and collection mode diameters of 200 and 84 μm in the crystal, respectively. With these parameters, we achieved a typical pair detection efficiency of 40% measured with standard single-photon avalanche diodes (SPADs), whose detection efficiency was estimated to be 50% at 820 nm, implying a collection efficiency of 80%. Owing to the asymmetry of the steering task, the source and detection system do not have to be symmetric. For example, in our setup Alice does not employ narrow-band filters; this choice increases her overall background, but reduces her loss, thus increasing the detection efficiency conditioned on Bob's measurement. Another key requirement is high photon detection efficiency. The conditional detection probability η is upper bounded by the performance of Alice's photon detectors, and therefore would not even in a loss-less, noise-free case allow us to meet the requirements of equation (4) with our SPADs and two measurement settings; in our experiment, Alice thus employs highly efficient TESs [18] . These detectors utilize a layer of superconducting tungsten kept in the transition temperature range and offer a combination of photon number resolution and high detection efficiency of up to 95% at 1,550 nm, while being virtually free of dark counts [18] . Our detectors were optimized for 810 nm with an optical cavity similar to that presented in an earlier work [18] , with an estimated detection efficiency for 820 nm photon in the 1,550 nm single-mode SMF-28 fibre connected to this cavity to be larger than 97%. In practice, the measured detection efficiencies of our two TES were 1.50 and 1.56 times higher than the efficiency of our reference SPAD at 820 nm. The dominant source of optical loss, which leads to these less-than-optimal figures, was a splice between the single-mode 820-nm fibres connected to the source and the fibres connected to the TES, which were single mode at 1,550 nm. The TESs were operated between 40 and 75 mK and yielded analogue output pulses with a rise time of ∼ 320 ns and jitter of ∼ 78 ns. To detect coincidences between the TES signals and the TTL pulses generated by the SPADs, each amplified TES signal was digitized with a constant fraction discriminator. Because the TESs rethermalize with a relaxation period of ∼ 2 ms after each detection event, the non-number resolving discriminators were set to impose a dead time of the same length to avoid false detections. To match the delay caused by the TES detection system, Bob's SPAD signals were delayed by ∼ 450 ns. Coincident events were then detected with a field-programmable gate array with a timing window of 98 ns. The long dead time period imposed by our electronics leads to a rate-dependent loss and we therefore operated the source at comparatively low rates of photon-pair creation. We achieved optimal conditional detection efficiency at a laser pump power of 250 μW, generating ∼ 12 kHz of single photons in each TES channel. At this rate, the loss due to dead time was ∼ 2.5%. Experimental violation of our steering inequality We produced the polarization-entangled singlet state where | H 〉 and | V 〉 represent single horizontal and vertical polarized photons, respectively, and performed separate measurements in 2 and 3 different bases ( N =2, 3, with measurements of , Ŷ and Ẑ ). 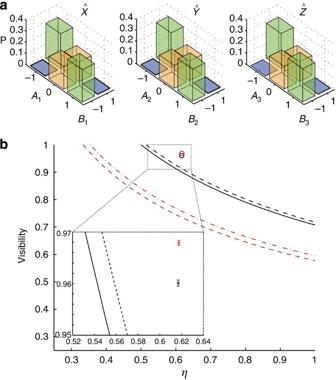Figure 3: Experimental violation of a steering inequality. (a) Probability distributionsP(Ai=a,Bj=b) for theS3measurements,ŶandẐcalculated by normalizing the registered coincident events for each measurement setting to the total count numbers. The green and blue bars represent correlations that indicate the quality of the shared entangled state. The orange bars represent events that Alice failed to detect. Error bars are too small to be seen on this scale. ForS2, we used the data obtained from the measurements ofandŶ. (b) Theoretical visibility required to violate steering inequalities forN=3 (red dashed line) andN=2 (black line) for a given efficiencyη. Our measurement clearly violates this bound, with an averaged visibility ofV=0.9678±0.0005 at a mean heralding efficiency ofη=0.6175±0.0008 for theN=3 measurements (red) andV=0.9601±0.0006,η=0.6169±0.0008 forN=2 (black). All error bars (1 s.d.) were calculated assuming Poissonian photon-counting statistics. The correction to the analytic bound of inequality (3) due to measurement imprecision (calculated in the Methods section) is shown by the dash-dotted red line forS3and the dashed black line forS2. The discrete probability distribution for Alice and Bob's correlations, P ( A i = a , B j = b ), is shown in Figure 3a . From these, we first estimated an averaged heralding efficiency η and entangled state visibility V and compared them to the theoretical minimum requirements, equation (4), in Figure 3b . The plot indicates a conclusive, detection-loophole-free demonstration of steering. Figure 3: Experimental violation of a steering inequality. ( a ) Probability distributions P ( A i = a , B j = b ) for the S 3 measurements , Ŷ and Ẑ calculated by normalizing the registered coincident events for each measurement setting to the total count numbers. The green and blue bars represent correlations that indicate the quality of the shared entangled state. The orange bars represent events that Alice failed to detect. Error bars are too small to be seen on this scale. For S 2 , we used the data obtained from the measurements of and Ŷ . ( b ) Theoretical visibility required to violate steering inequalities for N =3 (red dashed line) and N =2 (black line) for a given efficiency η . Our measurement clearly violates this bound, with an averaged visibility of V =0.9678±0.0005 at a mean heralding efficiency of η =0.6175±0.0008 for the N =3 measurements (red) and V =0.9601±0.0006, η =0.6169±0.0008 for N =2 (black). All error bars (1 s.d.) were calculated assuming Poissonian photon-counting statistics. The correction to the analytic bound of inequality (3) due to measurement imprecision (calculated in the Methods section) is shown by the dash-dotted red line for S 3 and the dashed black line for S 2 . Full size image Indeed, for the steering parameter S 3 defined in (3), we obtained where the uncertainty (1 standard deviation) was calculated by standard propagation of the Poissonian photon-counting statistics. The corrected bound, due to imprecision in Bob's measurements and as calculated in the Methods section, was 1.062±0.003. This corresponds to a violation of inequality (3) by more than 200 standard deviations. For N =2, the corresponding corrected bound of inequality (3) was 1.029±0.0019. We obtained the value for the experimental steering parameter, yielding a violation of the steering inequality by 48 standard deviations. Our highly efficient system allows us to firmly close the detection loophole in this demonstration of quantum steering, achieving the highest ever reported heralding efficiency for entangled photons, η ≈62%. The experimental violation of inequality (3) has a quite intuitive interpretation: it shows that Alice can, at her will, steer Bob's qubit state to be preferably polarized along any of the three axes of the Bloch sphere, as demonstrated in Figure 3a . While we have closed the detection loophole, we have not addressed the locality and freedom of choice loopholes [20] in this work; closing these would require Alice and Bob's choice and implementation of measurements to be space-like separated, as demonstrated in a very recent experiment reported in ref. 21 . For practical purposes in quantum communication, however, these loopholes are typically not problematic [22] : it is a necessary assumption that Alice and Bob can choose their measurements independently of the state preparation, and that no unwanted information leaks from Alice and Bob's laboratories. Besides the criteria employed here there are others that can be used to demonstrate steering [13] , [23] . If Alice cannot achieve the high heralding efficiencies obtained in our experiment, some of these may be advantageous: as recently shown in ref. 24 , generalizing the linear criteria of ref. 14 allows for steering with arbitrarily high losses. However, these require a larger number of different measurement settings up to N =16 in the experiment reported in ref. 23 . Our choice to test inequality (3) was motivated by its simplicity in how it naturally accounts for Alice's detection inefficiencies, and by its minimality in the number of settings. Note that N =2 is the number of settings initially discussed by EPR; it is also the canonical number of settings in applications to quantum cryptography [10] . Increasing Alice's detection efficiency above 65.9% will enable steering to be used for quantum key distribution where one party distrusts their apparatus [10] , [25] ; our experiment thus constitutes an important step towards practical applications of quantum steering. Furthermore, our results imply that a fully loophole-free photonic Bell test seems to be within arm's reach. While the symmetric photon pair detection efficiency for our setup is somewhat lower than the conditional detection probability η , it is not far below the limit required to violate a Clauser-Horne inequality [26] with non-maximally entangled states [27] . Although still a technological challenge, it is now conceivable to surpass this efficiency in the near future, while simultaneously addressing the locality and freedom-of-choice loopholes such as demonstrated in ref. 20 . Note that detection-loophole-free Bell experiments have already been performed in ionic [28] and solid-state [29] systems. These systems however present significant difficulties in reaching the required spatial separation to simultaneously close the locality loophole. Proof of inequality (3) Inequality (3) is equivalent to previously derived variance criteria [13] , [30] . For completeness, we give here a simple and self-contained proof. If the observed correlation can be explained by the source sending non-entangled states to Alice and Bob, then the probability distribution P can be decomposed in the form where λ describes the source preparation, used with probability q λ (such that q λ ≥0, —note that the sum could in principle be continuous and infinite): it specifies Alice's response function P λ ( A i = a ) implemented by her (untrusted) measurement device, and the state ρ λ sent to Bob. The trusted observable B̂ j , chosen and fixed by Bob, then generates Bob's response function as quantum mechanics predicts. From the above decomposition, and defining such that, as before, and we get and By the co-nvexity of the square, which leads to Now, for any 1-qubit state ρ λ , and for 3 mutually unbiased observables B̂ i , one has (due to an uncertainty relation [31] ) Together with the previous inequality and the normalization , we obtain inequality (3), for N =3; the case for N =2 follows trivially. The maximal violation of a steering inequality arises from the unbiased observables maximizing local uncertainty [31] , reducing the classical bound, while the measurement results at the two locations represent perfect steering of states, maximizing the quantum bound. Correcting for Bob's imperfect measurements In the steering protocol no assumption is made about Alice's measurement device, which therefore need not be carefully characterized. Inequality (3) is, however, highly dependent on Bob's measurements: it is only valid when Bob measures mutually unbiased observables on qubits. In a practical experiment, however, Bob will not measure along perfectly mutually unbiased bases, and his operators may not act on a two-dimensional system only. We show now that the parameter S N can still be used to demonstrate steering, but the upper bound in (3) must be adapted according to Bob's actual measurement. Let us start by giving a more accurate description of the measurement Bob performs in our experiment. First, he uses quarter- and half-wave plates, which define a direction (that is, a unit vector) on the Bloch sphere, representing his choice of basis. The beam displacer (BD) then separates the H and V polarizations: a fraction t ≃ 1 of the H polarization goes to its first output channel, and later on to the ''+1'' detector, while a fraction 1 − t ≪ 1 (in our experiment, 1 − t ≤ 10 −15 ) goes to the second output channel, and to the ''−1'' detector. We can assume that, symmetrically, a fraction t of the V polarization goes to the second output channel, while a fraction 1− t goes to the first output channel, as we utilize a calcite BD as our polarizing element; its intrinsic birefringence maps polarization into different spatial modes, which is a fundamentally symmetric effect [32] . Note that other polarizing elements require a slightly more thorough analysis. We finally denote by η + and η − the overall detection efficiencies of the +1 and −1 detectors (SPADs), respectively, including all losses in Bob's lab, including coupling and detection losses. For a single-photon state entering Bob's lab, represented by a vector in the Bloch sphere, the probability that it gives a click on the +1 or −1 detector is then It follows that and with Hence, defining we get and by convexity, Consider now N =2 or 3 measurement directions , such that for all i ≠ j , for some ɛ >0 quantifying the non-orthogonality of the N directions. One can show that for all in the Bloch sphere, Indeed the worst case is obtained when the N vectors are such that for all i ≠ j , and when is a unit vector equidistant to the , which gives the upper bound above. Following the proof of inequality (3), we now obtain, for Bob's actual measurements, the steering inequality In our experiment, the ratio of detection efficiencies in Bob's two detectors was We estimated the orthogonality ɛ of Bob's measurements by inserting a large ensemble of different linear polarization states into Bob's measurement device, fully characterizing the two wave-plates and the relative coupling. For the N =3 measurement settings, we can take epsilon to be the maximum of all three scalar products we found in that case. For the test with N =2 settings, we used the two most orthogonal settings, and Ŷ , which gave From (5), this yields bounds of 1.0291±0.0019 and 1.062±0.003 for S 2 and S 3 , respectively, as quoted in the main text. Other experimental imperfections include dark counts and background of the detectors at tens of hertz, compared with a rate of ∼ 12 kHz total detected events for Bob. These will however only introduce some white noise into Bob's data, and cannot increase the bound in the steering inequality. The previous calculations assumed that Bob received qubit states, encoded in the polarization of single photons. This is however not guaranteed, and the source could indeed send multiphoton states. This problem can be treated if it is assumed that Bob has perfectly orthogonal measurements, linear detectors with equal efficiencies and randomly assigns outcomes for measurements with multiple detections. Indeed, using a squashing operation [33] —which maps a larger Hilbert space into a qubit space—it can be shown that treating the outputs of our measurements as representing qubit states will in no cases allow a state without bipartite entanglement to violate steering inequality (3). Although it is not straightforward to extend the results of ref. 33 to imperfectly orthogonal measurements, intuitively it is clear that the assignment of random outcomes to multiple detection events will reduce Alice and Bob's correlations, and will not help Alice's untrustworthy devices to increase the steering parameter S N . This intuition holds even if the detector efficiencies are not balanced, accounted for in our treatment of imprecise measurements, inequality (5). Given this, in the experiment Bob assigned a random outcome to the 0.07% of events that were double clicks. It is an open question whether squashing could also to some extent account for more realistic detectors with potential nonlinear response [34] . This effect—and other detector imperfections—could potentially be exploited by an untrusted party [35] . While these attacks are not an issue for a laboratory steering test similar to ours, they should definitely be considered in the design of any real-world quantum communication scheme, including future ones relying on steering inequalities. How to cite this article: Smith, D. H. et al . Conclusive quantum steering with superconducting transition-edge sensors. Nat. Commun. 3:625 doi: 10.1038/ncomms1628 (2012).